Optical detection of a single rare-earth ion in a crystal Rare-earth-doped laser materials show strong prospects for quantum information storage and processing, as well as for biological imaging, due to their high-Q 4 f ↔4 f optical transitions. However, the inability to optically detect single rare-earth dopants has prevented these materials from reaching their full potential. Here we detect a single photostable Pr 3+ ion in yttrium aluminium garnet nanocrystals with high contrast photon antibunching by using optical upconversion of the excited state population of the 4 f ↔4 f optical transition into ultraviolet fluorescence. We also demonstrate on-demand creation of Pr 3+ ions in a bulk yttrium aluminium garnet crystal by patterned ion implantation. Finally, we show generation of local nanophotonic structures and cell death due to photochemical effects caused by upconverted ultraviolet fluorescence of praseodymium-doped yttrium aluminium garnet in the surrounding environment. Our study demonstrates versatile use of rare-earth atomic-size ultraviolet emitters for nanoengineering and biotechnological applications. Apart from being the cornerstone of modern laser technology, crystals and glasses doped with rare-earth metals are known to have excellent properties for classical and quantum information storage and for performing quantum computation protocols [1] , [2] , [3] , [4] , [5] . They historically set the performance mark for these applications. Examples include demonstrations of optical memory in europium-doped yttrium silicate (Eu:YSO) [1] , two-qubit gates in Eu:YSO (ref. 2 ), storage of quantum coherence in Pr 3+ :YSO for over a second [3] , single photon storage in Nd 3+ :YVO 4 (ref. 4 ), preservation of entanglement after photon storage and readout in Nd 3+ :YSO (ref. 5 ), etc. Another rapidly developing field of research on rare-earth-doped optical materials is creation of photostable upconverting multicolour fluorescent markers for bioimaging with low background [6] , [7] . While quantum applications of rare-earth-doped materials take advantage of the high quantum efficiency of their high quality-factor optical transitions in a solid as well as the numerous optical Raman transitions suitable for spin–photon entanglement, biological applications benefit from the complex energy level structure of rare-earth ions, their exceptional photostability, long lifetimes of the excited electronic states and high flexibility in choosing the dopant species and host material. Long fluorescent lifetimes of 4 f ↔ 4 f transitions of rare-earth emitters result in their low emission rate and, consequently, inability to detect a single ion. At the same time, such detection would be highly beneficial for both quantum, biological and nanophotonic applications resulting in a fully functional rare-earth-based qubit with exceptionally long coherence lifetime [8] and, on the other hand, ultimately small photostable fluorescent biomarker [9] and versatile nanoscopic light source for near field microscopy or biomanipulation. Only a very limited number of indirect observations of a few rare-earth impurities have been reported due to their low fluorescence yield [10] , [11] , [12] . However, the emission rate of rare-earth centres can be dramatically improved by promoting the ions into higher-lying electronic states from which they can emit more efficiently due to much stronger low-Q parity-allowed transitions between 4 f n− 1 5 d excited and 4 f n ground states. In that way, the excitation–emission cycle shortens by orders of magnitude, whereas the fluorescence yield increases by the same factor. Here we demonstrate optical detection of a single rare-earth ion, namely, trivalent praseodymium, in a crystalline host (in the present case, yttrium aluminium garnet, YAG). We exploit the visible-to-ultraviolet upconversion phenomenon in Pr 3+ :YAG [13] to boost the efficiency of excitation–emission cycle and make a single Pr 3+ ion detectable. High-quality photon antibunching measurements prove that the emission originates from a single quantum object, whereas excitation spectra and their polarization dependence prove that the single emitter is indeed a Pr 3+ ion. The same approach can be used to detect Pr 3+ in other hosts including low-spin YSO [14] in which decoherence time of the dopant nuclear spin is the longest [8] . We also show that the ultraviolet emission originating from Pr 3+ in YAG under visible excitation induces photochemical effects in the surrounding environment, such as exposure of photoresists and apoptotic cell death. Optical properties of Pr 3+ :YAG YAG has a complex crystal structure with yttrium ions occupying distorted octahedral sites of D 2 symmetry as shown in Fig. 1a and b . Praseodymium dopant ions substitute yttrium in these sites. The electronic level structure of Pr 3+ ion in YAG crystal is well studied [15] . It is represented by a number of 4 f 2 states of rather low energy and more energetic 4 f 5 d states as depicted in Fig. 1c,d . 4 f 2 states are formed by the combined action of the central Coulomb potential of the [Xe] core of Pr 3+ , Coulomb interaction of the unpaird 4 f electrons, spin–orbit coupling and crystal field potential. All states belong to either of the four irreducible representations Γ 1−4 of the symmetry group D 2 . The ground state of Pr 3+ is the 3 H 4 multiplet split by crystal field into nine sublevels. 4 f 2 states of higher energy give rise to spectrally narrow parity forbidden optical transitions in the visible and infrared. Higher lying electronic levels belonging to the 4 f 5 d shell give rise to parity allowed optical transitions to 4 f 2 states. The 5 d electron is not screened from its crystalline environment by outer 5 s 2 and 5 p 2 shells as in the case of 4 f electrons. Therefore, 4 f 2 ↔ 4 f 5 d transitions exhibit strong phonon sidebands in absorption and emission similar to singlet–singlet optical transitions in organic dyes or triplet–triplet transitions in nitrogen-vacancy centre in diamond [16] . Higher lying 4 f 5 d states suffer from radiationless decay into the lowest 4 f 5 d level from where fluorescence emission commences. Emission originating from this level covers a spectral range 300–450 nm [17] . The quantum efficiency of this ultraviolet transition is close to unity even at room temperature [18] with lifetime ≈18 ns. Thus, ultraviolet fluorescence can be used for detecting a single Pr 3+ ion in a YAG crystal. It can be excited either by direct ultraviolet (shorter than 300 nm) pumping into the absorption phonon sidebands of 4 f 5 d levels or by a two-step upconversion excitation process involving an intermediate 4 f 2 state. The second way of exciting Pr 3+ is more advantageous for a number of reasons. First of all, excitation with wavelengths shorter than 300 nm would inevitably produce strong fluorescent background from the optical elements along the excitation path (mainly the focusing objective lens) within the detection range (300–450 nm). Second and most importantly, the two-step pumping allows one to exploit the spectrally narrow features of the 4 f 2 ↔4 f 2 transitions in the first pumping step and read out the result of the manipulation with the second pumping step. 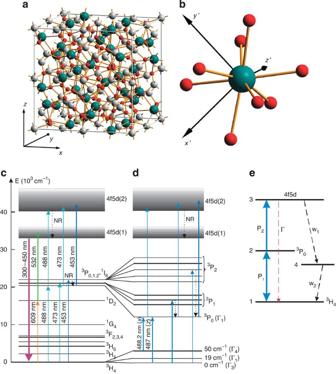Figure 1: Optical properties of Pr3+ion in YAG. (a) Unit cell of YAG crystal. Green, white and red sites are occupied by yttrium, aluminium and oxygen, respectively. All together, the unit cell contains eight molecular units Y3Al5O12. Praseodymium occupies yttrium sites substitutionally. (b) The local surrounding of one yttrium site. The orientation is identical to (a). While the localz′-axis is along theycrystal axis, the axesx′ andy′ are rotated with respect toxandzcrystal axes by 45°. Other five local symmetries can be obtained from this one by one or two successive 90° rotations aroundx,yandzcrystal axes. (c) Electronic level structure of Pr3+ion in a YAG crystal. Relevant optical transitions are indicated by arrows. NR, non-radiative decay channels. (d) Fine structure of3H4→3P0,1,2transitions giving rise to upconverted ultraviolet fluorescence. Only the lowest three sublevels of3H4manifold populated at room temperature are shown. (e) Four-level model used to explain the shape of photon antibunching signal. The metastable trapping state is assumed to be populated via decay of the emitting state 3. Figure 1: Optical properties of Pr 3+ ion in YAG. ( a ) Unit cell of YAG crystal. Green, white and red sites are occupied by yttrium, aluminium and oxygen, respectively. All together, the unit cell contains eight molecular units Y 3 Al 5 O 12 . Praseodymium occupies yttrium sites substitutionally. ( b ) The local surrounding of one yttrium site. The orientation is identical to ( a ). While the local z ′-axis is along the y crystal axis, the axes x ′ and y ′ are rotated with respect to x and z crystal axes by 45°. Other five local symmetries can be obtained from this one by one or two successive 90° rotations around x , y and z crystal axes. ( c ) Electronic level structure of Pr 3+ ion in a YAG crystal. Relevant optical transitions are indicated by arrows. NR, non-radiative decay channels. ( d ) Fine structure of 3 H 4 → 3 P 0,1,2 transitions giving rise to upconverted ultraviolet fluorescence. Only the lowest three sublevels of 3 H 4 manifold populated at room temperature are shown. ( e ) Four-level model used to explain the shape of photon antibunching signal. The metastable trapping state is assumed to be populated via decay of the emitting state 3. Full size image There are a number of processes that can lead to upconverted ultraviolet emission of Pr 3+ in YAG as shown in Fig. 1c,d . The first one is excitation of a metastable 1 D 2 state with an orange laser (611 or 609 nm) followed by the second excitation step at 532 nm. This method was used by us to demonstrate super-resolution microscopy of Pr:YAG nanoparticles [19] . Even a single colour optical pumping in the orange can be used though this upconversion scheme is much less efficient [17] . The second and the most straightforward way being exploited in the present work is to use 3 H 4 ↔ 3 P 0,1,2 transitions as the first upconversion step [13] . Once promoted into 3 P 0 state, the electron can be excited further into 4 f 5 d (2) band, nonradiatively decay onto the emitting 4 f 5 d (1) level, and emit an ultraviolet photon. As will be shown below, this results in a number of sharp (>1 nm at room temperature) upconversion resonances whose width is determined by the first excitation step. A simplified level structure diagram showing upconversion process via 3 P 0 state is given in Fig. 1e . This model will be used later for description of Pr 3+ excited-state dynamics. Localization of a single Pr 3+ ion in YAG Praseodymium is one of the most abundant impurities in yttrium-based compounds [20] . To localize a single Pr 3+ ion in a bulk YAG crystal, the distance between the neigbouring praseodymium ions must be greater than the resolution of the optical setup. This sets the upper limit of 1 ppb (parts per billion) on the praseodymium dopant concentration relative to yttrium. As we show below, the purest commercially available YAG crystals satisfy this condition. At cryogenic temperatures the requirements on the crystal purity can be significantly relaxed by spectrally selecting a subensemble of ions within an inhomogeneous excitation profile by means of a narrow-band excitation laser [21] , [12] . However, a much simpler approach towards isolation of a single Pr 3+ impurity even at room temperature is to use Pr-doped YAG nanoparticles finely dispersed on a substrate (see Methods section). Samples prepared in this way were optically studied in a home-built high-resolution fluorescent microscope (see Methods section for details on its construction). A fluorescent image of nanoparticles is shown in Fig. 2a . Most of the bright spots on the image reveal several (up to 20–30) Pr 3+ centres and are thought to be clusters of nanoparticles. However, the antibunching measurements performed on the marked nanoparticles revealed g (2) function, indicating single photon emission from those particles. 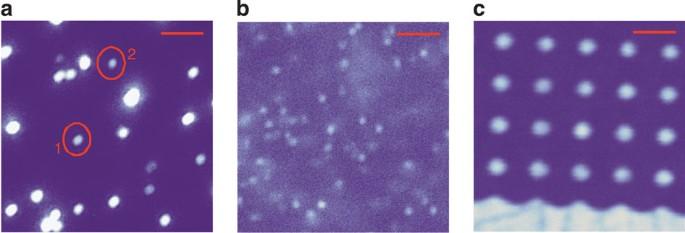Figure 2: Upconversion scanning microscopy images of Pr3+:YAG. (a) Ultraviolet fluorescence image of YAG nanoparticles dispersed on a glass slide. Within the 10×10 μm2scan two marked spots are showing single emitter antibunching. (b) Fluorescence image of high purity YAG crystal. Bright spots are attributed to individual Pr3+single ion impurities. (c) Ultraviolet fluorescence image of nominally pure YAG single crystal implanted with Pr3+ions. The implantation mask contained holes arranged in a square grid. Scale bars in all three panels correspond to 2 μm. Figure 2: Upconversion scanning microscopy images of Pr 3+ :YAG. ( a ) Ultraviolet fluorescence image of YAG nanoparticles dispersed on a glass slide. Within the 10×10 μm 2 scan two marked spots are showing single emitter antibunching. ( b ) Fluorescence image of high purity YAG crystal. Bright spots are attributed to individual Pr 3+ single ion impurities. ( c ) Ultraviolet fluorescence image of nominally pure YAG single crystal implanted with Pr 3+ ions. The implantation mask contained holes arranged in a square grid. Scale bars in all three panels correspond to 2 μm. Full size image A high purity YAG crystal was also searched for single Pr 3+ emitters. A typical fluorescent image of the sample is shown in Fig. 2b . In the present 10×10 μm 2 scan around 60 individual ions are seen. With the measured depth resolution being 1 μm, we estimate the density of praseodymium impurities to be 6×10 11 cm −3 or 0.04 ppb relative to yttrium. Unlike nanoparticle sample, the out-of-focus Pr 3+ impurities caused significant background fluorescence contributing to 35% of the signal. Therefore, the photon antibunching deep corresponding to a single emitting centre had only ≈30% contrast and was rather noisy ( Supplementary Fig. S1 ). Furthermore, the fluorescent signal collected from individual Pr 3+ ions in the bulk crystal was 2.5 times lower compared with the nanoparticle case. All experiments described below in this section are thus carried out on single praseodymium ions in YAG nanocrystals. Spectral properties of a single Pr 3+ in YAG The photon antibunching signal from a single Pr 3+ ion is shown in Fig. 3a . Owing to the upconversion process, the fluorescent background (~100 counts s −1 ) is negligible compared with the signal from the single emitting centre (~1.3×10 4 counts s −1 ). Centres are usually photostable at room temperature for many hours of continuous illumination. To prove that fluorescence is indeed from a Pr 3+ ion in YAG host, the excitation spectrum of upconverted fluorescence was measured and the results are shown in Fig. 4a–c . The spectra exactly match previously reported experimental results on Pr:YAG visible-to-ultraviolet upconversion [13] , absorption spectra of Pr 3+ :YAG (ref. 22 ), and our own measurements performed on a bulk YAG crystal doped with 0.18% of Pr 3+ . They consist of a number of sharp (down to <0.5 nm) lines and exemplify the high spectral selectivity of the upconversion process even at room temperature. Further evidence for Pr 3+ excitation comes from the polarization selectivity of the first upconversion step. The optical dipoles associated with transitions between any states of Γ m and Γ n symmetry representations are oriented along the principal axes of the local dodecahedron [15] as indicated in Fig. 1b : Γ 1 ↔Γ 4 and Γ 2 ↔Γ 3 are along x -axis, Γ 3 ↔Γ 4 and Γ 1 ↔Γ 2 are along y -axis, and Γ 1 ↔Γ 3 and Γ 2 ↔Γ 4 are along z -axis. The transitions Γ n ↔Γ n between the states of the same group representation are forbidden. At room temperature only 3 out of 9 sublevels of lowest energy belonging to 3 H 4 manifold, namely, Γ 3 (0 cm −1 ), Γ 1 (≈19 cm −1 ) and Γ 4 (≈50 cm −1 ), are populated. Thus, for example, in the vicinity of 3 H 4 → 3 P 0 (Γ 1 ) transition the two allowed optical dipoles, Γ 3 ( 3 H 4 )→Γ 1 ( 3 P 0 ) (487.0 nm) and Γ 4 ( 3 H 4 )→Γ 1 ( 3 P 0 ) (488.2 nm) (corresponding transitions are indicated in Fig. 1d ), should have z - and x -orientations, respectively. Same arguments apply to 3 H 4 → 3 P 1,2 excitations. Polarization dependence of the excitation spectra are shown in Fig. 4d–f and reveal the projections of the x and z dipoles onto the plane of the sample. For the ion investigated, we could not identify the direction of the y dipole at room temperature. The probable reason for this is that y -polarized transitions are much weaker than x and z ones. Qualitatively similar results were obtained for other spots indicating single photon emitter behaviour. Overall, 39 single upconverting emitters were found within a 100×100 μm 2 area. Statistical analysis of their excitation line positions in the vicinity of 3 H 4 → 3 P 0 transition is shown in Supplementary Fig. S2 . 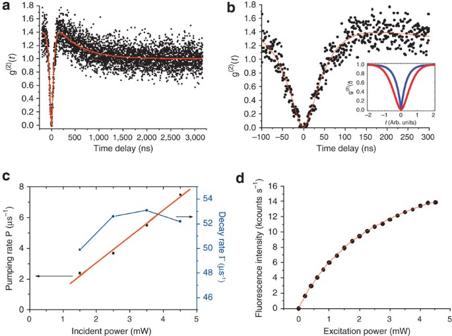Figure 3: Excited-state dynamics of a single Pr3+ion. (a) Normalizedg(2)function measured at spot 1 onFig. 2awith 4.5 mW of excitation at 488.2 nm wavelength. The signal is fitted with the solution of the rate equations according to the four-level model shown inFig. 1e(red line). (b) Zoom into zero-delay region of the antibunching curve. Flat bottom corresponding to quadratic temporal dependence is clearly seen. The inset compares the theoretical antibunching shapes of the emissions originating from one-step (blue, casp-like) and two-step (red, parabolic at the bottom) excitations. (c) Power dependences of the pumping rateP(black squares) and radiative decay Γ (blue circles) extracted from the fits of antibunching signals taken at 1.5, 2.5, 3.5 and 4.5 mW are shown. Taking the focused laser spot diameter to be ≈300 nm (the size of the nanoparticle seen by our microscope) and specified 85% transmission of the objective lens in the range 480–490 nm, the derived pumping rate gives the ground- and excited-state absorption cross-sections to be 7×10−19cm2. This value agrees well with ground-state absorption cross-section of 6×10−19cm2deduced from the data reported previously33and with excited-state absorption cross-section of 8×10−19cm2(ref.23) for 532 nm wavelength. (d) Saturation behaviour of ultraviolet fluorescence at spot 1. Saturation power is 2.75 mW, whereas saturated fluorescence count rate is 22.5 kcounts s−1. Figure 3: Excited-state dynamics of a single Pr 3+ ion. ( a ) Normalized g (2) function measured at spot 1 on Fig. 2a with 4.5 mW of excitation at 488.2 nm wavelength. The signal is fitted with the solution of the rate equations according to the four-level model shown in Fig. 1e (red line). ( b ) Zoom into zero-delay region of the antibunching curve. Flat bottom corresponding to quadratic temporal dependence is clearly seen. The inset compares the theoretical antibunching shapes of the emissions originating from one-step (blue, casp-like) and two-step (red, parabolic at the bottom) excitations. ( c ) Power dependences of the pumping rate P (black squares) and radiative decay Γ (blue circles) extracted from the fits of antibunching signals taken at 1.5, 2.5, 3.5 and 4.5 mW are shown. Taking the focused laser spot diameter to be ≈300 nm (the size of the nanoparticle seen by our microscope) and specified 85% transmission of the objective lens in the range 480–490 nm, the derived pumping rate gives the ground- and excited-state absorption cross-sections to be 7×10 −19 cm 2 . This value agrees well with ground-state absorption cross-section of 6×10 −19 cm 2 deduced from the data reported previously [33] and with excited-state absorption cross-section of 8×10 −19 cm 2 (ref. 23 ) for 532 nm wavelength. ( d ) Saturation behaviour of ultraviolet fluorescence at spot 1. Saturation power is 2.75 mW, whereas saturated fluorescence count rate is 22.5 kcounts s −1 . 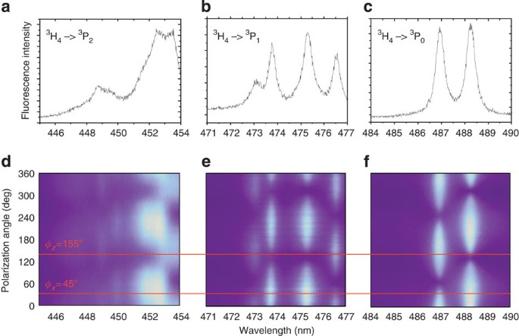Figure 4: Spectral properties of a single Pr3+ion. (a–c) Excitation spectrum of ultraviolet emission from centre 1 onFig. 1ain the vicinity of3H4→3P2,3H4→3P1and3H4→3P0transitions, respectively. (d–f) show the dependence of the corresponding spectra on the polarization of the excitation beam. Full size image Figure 4: Spectral properties of a single Pr 3+ ion. ( a – c ) Excitation spectrum of ultraviolet emission from centre 1 on Fig. 1a in the vicinity of 3 H 4 → 3 P 2 , 3 H 4 → 3 P 1 and 3 H 4 → 3 P 0 transitions, respectively. ( d – f ) show the dependence of the corresponding spectra on the polarization of the excitation beam. Full size image Excited-state dynamics The fluorescence lifetime measurements performed on spot 1 with frequency-doubled femtosecond Ti:sapphire laser operating at 906 nm (453 nm for the doubled output) revealed 19 ns in rather good agreement with known value of 18 ns lifetime of the lowest 4 f 5 d state of Pr 3+ ion in YAG. The saturation behaviour of Pr 3+ fluorescence as a function of excitation intensity at 488.2 nm is shown in Fig. 3d . Three fluorescent regimes are expected: quadratic dependence at very low excitation power; linear dependence once the transition 3 H 4 ↔ 3 P 0 is saturated while the second step is not; and full saturation. The absorption cross-sections from the ground state 3 H 4 to the intermediate 3 P 0 and the one from 3 P 0 to 4 f 5 d (2) are approximately identical, ~6–8×10 −19 cm 2 (ref. 23 ), but the intermediate and the emitting states have significantly different lifetimes, 8 μs and 18 ns, respectively. Only linear and fully saturated regimes were observed experimentally as saturation of the first excitation step occurs at very low excitation intensity at which no upconverted ultraviolet fluorescence was possible to collect. The shape of the photon correlation signal reveals two distinct features: significant bunching at non-zero time delays and very flat bottom of the antibunching dip, clearly visible in Fig. 3b . The former indicates the existence of a metastable state, which can effectively trap population for rather a long time [24] . Probable candidates for this metastable state are the 1 G 4 level whose lifetime is known to be ≈0.4 μs (ref. 25 ), the very long-lived 1 D 2 level, which, however, can be repumped by the excitation laser, the 3 H 4 and 3 H 5 levels of unknown lifetime or some electron trap within the YAG bandgap. The latter can be populated by ionization of Pr 3+ due to excited-state absorption from the emitting 4 f 5 d (1) level [23] . A simplified 4-level model depicted in Fig. 1e is used to describe the second feature of the g (2) ( t ) function. The Pr 3+ ion is pumped from its ground state 1 ( 3 H 4 ) into an intermediate state 2 ( 3 P 0 ) and back at rate P 1 . From state 2 it can be promoted further into state 3 (4 f 5 d ) at pumping rate P 2 from where it can decay either into level 1 at rate Γ emitting an ultraviolet photon or into a metastable state 4 at rate w 1 . Finally, the metastable state can decay into level 1 at rate w 2 . After the start photon is detected by the Hanbury–Brown and Twiss setup, the initial populations of the levels are ρ 11 (0)=1, ρ 22 (0)= ρ 33 (0)= ρ 44 (0)=0. The g (2) ( t ) function is determined as follows: At short time delays between start and stop photons, g (2) can be approximated as: The t 2 dependence of the intensity correlation function is an indication of probing the population of intermediate state 2 with the second excitation photon and explains the flat bottom of the antibunching dip. It can also be seen that the antibunching width is no longer approaching the lifetime of the emitting state for low pump power as in the case of a single-step excitation, but increases as ( P 2 +2 P 1 ) −1 . Under the assumption of equal pump rates P 1 = P 2 = P (in agreement with known absorption cross-sections) it is possible to fit the experimental antibunching curves with the numerical solutions of the set of rate equations and extract the pumping rates and decay parameters of the Pr 3+ ion as a function of pump intensity ( Fig. 3c ). The measured antibunching curves are shown in Supplementray Fig. S3 . As expected, the pumping rate increases linearly whereas the radiative decay rate Γ stays constant around 52 μs −1 . The latter value is in good agreement with the measured lifetime of ~19 ns. Implantation of Pr 3+ into YAG crystal Not only the ability to detect, but also to create fluorescent centres at the desired location in the crystal is a significant ingredient for the technological implementation of single Pr 3+ . We demonstrate that Pr 3+ centres can be created in pure bulk YAG crystals by ion implantation. Some parts of the surface of nominally pure YAG crystal were covered with photoresist with lithographically defined holes. After implantation the photoresist was removed and the sample was annealed at 1,200 °C. Figure 1c shows the upconverted fluorescence scan of the crystal surface subject to such patterned implantation with 30 keV praseodymium ions with an implantation dosage of 10 13 cm −2 . The grid of the holes in the photoresist is clearly seen. The excitation spectrum taken on the implanted region in the vicinity of 3 H 4 → 3 P 0 transition of Pr 3+ was similar to Fig. 4c, indicating that implantation was successful. However, the unimplanted area showed the same excitation spectrum though of 100 times lower brightness. This shows that the nominally pure crystal contained significant amount of optically unresolvable Pr 3+ impurities (the crystal used for implantation was much less pure than the one shown in Fig. 2 ). It is known from optical free-induction decay [26] , Raman-heterodyne [27] , and electromagnetically induced transparency [3] experiments that Pr 3+ ions in various hosts possess nuclear spin–flip optical Raman transitions. Once detected at cryogenic temperature, single fluorescent Pr 3+ ions would present a perfect qubit with all-optical access to its nuclear spin states possessing lifetimes of the order of tens of seconds [8] . In addition, lifetime-limited linewidth of optical transitions [28] and their 100% quantum efficiency would allow for efficient dipole–dipole optical coupling between praseodymium ions separated by as far as a few tens of nanometres in the same way as was demonstrated for dye molecules [29] . In turn, several mutually coupled praseodymium ions would comprise a multi-qubit quantum gate [2] while dipolar coupling to other rare-earth species would allow to use Pr 3+ as a readout qubit in rare-earth-based quantum computer designs [30] . However, cryogenic experiments with single Pr 3+ ions have to be carefully designed to maximize collection efficiency of ultraviolet fluorescence. In the present case, <2% of the emitted photons are being detected. More details on the estimate of the collection efficiency of the setup are given in Supplementary Methods . Implementation of solid immersion lenses (SILs) and dielectric antennas [31] could improve the situation. At the same time, proper identification of the metastable trapping state would show the way towards its repumping and, therefore, fluorescence efficiency increase. Apart from new opportunities for quantum computing, having a single photostable upconverting ultraviolet emitter at hand enables optical nano-engineering due to ultraviolet-triggered photochemical reactions in the surrounding of the emitter. For example, ultraviolet emission of a Pr:YAG nanoparticle can expose the surrounding photoresist. As the emission of a nanoparticle containing many Pr 3+ centres is isotropic, the nanoparticle lying on the substrate and covered with negative-tone photoresist will create a hemispherical shell for itself as illustrated in Fig. 5a . Such a self-assembled SIL will enhance the collection efficiency of the light emitted by this specific nanoparticle as it is situated in the very centre of the hemisphere. Experimental details of creation of a SIL are given in Supplementary Methods . The reconstructed atomic force microscopy image of such a self-assembled SIL is shown in Fig. 5b . The evaluation of SIL performance indicated 5–8 times enhancement in ultraviolet light collection efficiency as indicated in Supplementary Table S1 . This example demonstrates applicability of upconverting ultraviolet emission from rare-earth-doped materials for micro- and nanolithography, potentially, at a single-emitter level. This ultraviolet emission can also have biological effects. Although at low excitation power upconverted ultraviolet fluorescence can be used for bioimaging ( Supplementary Fig. S4 ), at higher fluences it can be used for site-specific cell degradation. To demonstrate that we cultured HeLa cells on the surface of bulk Pr:YAG crystal (0.18% Pr 3+ ). Subsequently, part of the crystal was illuminated by scanned focused laser beams of 532 and 609 nm wavelengths (this combination produces upconverted ultraviolet fluorescence according to Fig. 1c ). After illumination and incubation of the sample for 1 h, >50% of the cells in the irradiated region died ( Fig. 5c ), whereas the control region showed <10% of dead cells ( Fig. 5d ). Pr-doped nanocrystals thus present the opportunity of performing tightly localized (potentially, down to a few nanometers) photochemical reactions in living cells. 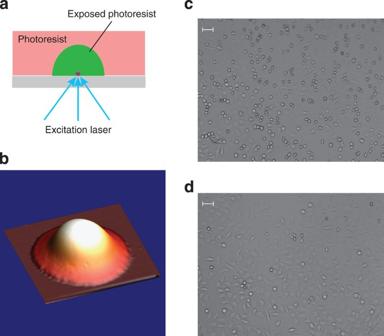Figure 5: Photochemical effects due to upconverted ultraviolet fluorescence. (a) Self-assembly of a SIL by isotropic exposure of negative-tone photoresist with ultraviolet emission of a nanoparticle. (b) Reconstructed 3D atomic force microscopy (AFM) image of a self-assembled SIL. Lateral size of the image is 6.6×6.6 μm2. (c) Light microscope image of HeLa cells on the surface of Pr:YAG crystal exposed by a combination of 609+532 nm lasers. Most of the cells died (round shaped). (d) Image of the cells exposed by a combination of wavelengths 600+532 nm (no upconverted ultraviolet is produced). Most of the cells are alive. The same fraction of live cells is found in the unexposed region. Scale bars on (c,d) correspond to 50 μm. Figure 5: Photochemical effects due to upconverted ultraviolet fluorescence. ( a ) Self-assembly of a SIL by isotropic exposure of negative-tone photoresist with ultraviolet emission of a nanoparticle. ( b ) Reconstructed 3D atomic force microscopy (AFM) image of a self-assembled SIL. Lateral size of the image is 6.6×6.6 μm 2 . ( c ) Light microscope image of HeLa cells on the surface of Pr:YAG crystal exposed by a combination of 609+532 nm lasers. Most of the cells died (round shaped). ( d ) Image of the cells exposed by a combination of wavelengths 600+532 nm (no upconverted ultraviolet is produced). Most of the cells are alive. The same fraction of live cells is found in the unexposed region. Scale bars on ( c , d ) correspond to 50 μm. Full size image Microscope and laser source construction Microscopic studies of Pr:YAG nanoparticles spin-coated on a glass slide were performed in a home-built scanning microscope shown schematically in Supplementary Fig. S5a and consisting of a 3D nanopositioning stage, a 425 nm shortpass dichroic beamsplitter, a high NA (1.30) oil immersion objective lens having high transmission in the UV (Zeiss Fluar UV), UV-transmitting filter (UG11 optical glass), UV 50/50 beamsplitter and two UV-sensitive single photon counting PMTs (Hamamatsu) to form a Hanbury–Brown and Twiss setup. Home-made tunable diode lasers with Littmann external cavity operating around 488 nm ( 3 H 4 ↔ 3 P 0 transition), 473 nm ( 3 H 4 → 3 P 1 transition) and 450 nm ( 3 H 4 ↔ 3 P 2 transition) were used as excitation sources (all diodes are from Nichia Corporation). The output of the diode lasers was passed through a single-mode optical fiber to assure Gaussian shape of the excitation beam. The illumination of the sample and the fluorescence collection were arranged through the same objective lens. Typical power of the excitation beam at the apperture of the objective lens was several milliwatts. Laser diode tuning Laser diodes were tuned by means of Littmann external cavity with 60° prism being a dispersion element as shown in Supplementary Fig. S5b . Single transverse mode laser diodes (488, 473 and 450 nm) were used as manufactured, that is without applying an antireflective coating on their output facets. Laser diode output collimated by an aspheric lens was dispersed by a prism. The first reflection from the dispersion prism was taken as an output beam. The tuning mirror was mounted on a tip-tilt piezo-driven mirror mount for automated wavelength tuning. Typical output power of the diode laser was in the range of a few tens of milliwatts with a possibility of tuning through 7 nm spectral range for 488 and 473 nm diodes and 11 nm spectral range for 450 nm diode. The linewidth of such a tunable laser source was below 0.1 nm. Nanoparticle preparation and characterization Pr-doped YAG nanocrystals exploited in the present work were prepared by a sol–gel pyrolysis method according to slightly modified procedure reported in work [32] . Praseodymium nitrate was added according to required stoichiometry aiming at dopant concentration of 2 ppm. Characterization of nanoparticles by X-ray diffraction measurements resulted in 32 nm average size of single crystalline YAG. Nanoparticles were spin-coated on a 150 μm-thick glass slide out of isopropanol suspension. X-ray diffraction spectrum and SEM image of YAG nanoparticles dried on silicon substrate are shown in Supplementary Figs S6 and S7 . How to cite this article: Kolesov, R. et al . Optical detection of a single rare-earth ion in a crystal. Nat. Commun. 3:1029 doi: 10.1038/ncomms2034 (2012).